Natural occurring epialleles determine vitamin E accumulation in tomato fruits Vitamin E (VTE) content is a low heritability nutritional trait for which the genetic determinants are poorly understood. Here, we focus on a previously detected major tomato VTE quantitative trait loci (QTL; mQTL 9-2-6 ) and identify the causal gene as one encoding a 2-methyl-6-phytylquinol methyltransferase (namely VTE3 (1)) that catalyses one of the final steps in the biosynthesis of γ- and α-tocopherols, which are the main forms of VTE. By reverse genetic approaches, expression analyses, siRNA profiling and DNA methylation assays, we demonstrate that mQTL 9-2-6 is an expression QTL associated with differential methylation of a SINE retrotransposon located in the promoter region of VTE3 (1). Promoter DNA methylation can be spontaneously reverted leading to different epialleles affecting VTE3 (1) expression and VTE content in fruits. These findings indicate therefore that naturally occurring epialleles are responsible for regulation of a nutritionally important metabolic QTL and provide direct evidence of a role for epigenetics in the determination of agronomic traits. Genetic determinants of nutritional quality have long been studied in many important crops [1] , [2] , [3] , [4] , [5] . However, mechanisms linking the few identified genetic determinants to the end phenotypes are largely unknown. This is true for tocochromanols, a group of compounds exclusively produced in photosynthetic organisms [6] , [7] and that includes tocopherols and tocotrienols (termed vitamin E-VTE-), which have high nutritional value in the human diet. Tocopherols are the molecules that show the highest VTE activity [8] . These compounds consist of a polar chromanol head group (derived from homogentisate) and a prenyl lipophilic side chain, products of the plastidial shikimate and methylerythritol phosphate pathways, respectively. The first step for tocopherol synthesis is catalysed by homogentisate phytyl transferase (VTE2, EC 2.5. 1.-), which condenses phytyl 2P and homogentisate to yield 2-methyl-6-phytylquinol. From this precursor, the four naturally occurring forms are synthesized. While γ- and α-tocopherol are produced by the sequential activities of dimethyl-phytylquinol methyl transferase (VTE3, EC 2.1.1.-), tocopherol cyclase (VTE1, EC 5.3.-.-) and tocopherol C-methyl transferase (VTE4, EC 2.1.1.95); δ- and β-tocopherol synthesis, do not require VTE3 activity being formed merely by the action of the latter two enzymes ( Fig. 1a ) [9] . The role of tocopherols as lipid-soluble antioxidants is well documented for plants and humans and occurs by two mechanisms: (i) donation of a hydrogen atom to a highly reactive polyunsaturated fatty acid peroxyl radical thus preventing a chain reaction of lipid peroxidation and (ii) physically or chemically quenching singlet oxygen species, which damage many biological molecules including proteins, DNA, carbohydrates and polyunsaturated fatty acids [10] . Given that photosynthesis is a major source of singlet oxygen, this quenching mechanism plays an important role in the functional regulation of photosystem II with important implications in physiological responses to high light conditions, low temperature and osmotic stress [11] . 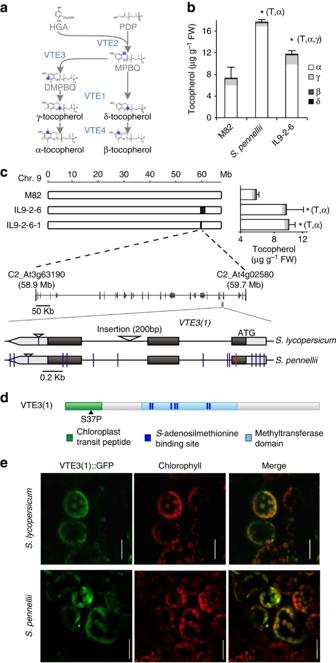Figure 1: Fine mapping of tocopherol QTL9-2-6. (a) The tocopherol core pathway in plants. Biosynthetic enzymes, homogentisate phytyl transferase (VTE2), dimethyl-phytylquinol methyl transferase (VTE3), tocopherol cyclase (VTE1) and γ-tocopherol C-methyl transferase (VTE4) are in blue types. Precursors and intermediates are: homogentisate (HGA), phytyl 2P (PDP), methyl-phytylquinol (MPBQ) and dimethyl-phytylquinol (DMPBQ). (b) Composition and total tocopherol contents (mean ±s.e.m,n=4) in ripe tomato fruits from the two parental species;S. lycopersicum(cv. M82) andS. pennellii(LA716), and the IL9-2-6 that shows the mapped QTL. (c) Fine mapping of the QTL9-2-6to a centromeric region of chromosome 9 harbouring the wild allele ofVTE3(1) gene. Through the analysis of 190 F2 and 50 F3 plants, derived from a cross between theS. lycopersicum(cv. M82) and the IL9-2-6, a recombinant subline (IL9-2-6-1) was obtained. Tocopherol contents (mean ±s.e.m,n=6) in ripe tomato fruits from these lines are shown on the right side of this panel. Genomic structure of the introgression contained in this line is shown below with black arrows indicating transcriptionally active genes. A magnified view ofS. lycopersicumandS. pennelliialleles ofVTE3(1) gene shows synonymous (blue bars) and non-synonymous (red bar) polymorphisms and insertions in the second intron and in the 3′UTR. Black and grey boxes represent exons and, 5' and 3' UTR, respectively. (d) Protein structure of the tomato VTE3(1) enzyme indicating the amino acid substitution (S37P). (e) Transient expression of both alleles of VTE3(1)::GFP fusion protein in mesophyll cells ofN. benthamianaleaves indicates chloroplast targeting under confocal microscopy examination. Asterisks in panelsbandcdenote statistically significant differences for total tocopherol (T) and the indicated tocopherol forms (t-testP<0.05). Scheme of chromosome 9 is based on physical distances calculated according to version SL2.4 of the tomato genome (www.solgenomics.net). White bar ineindicates 25 μm. Figure 1: Fine mapping of tocopherol QTL 9-2-6 . ( a ) The tocopherol core pathway in plants. Biosynthetic enzymes, homogentisate phytyl transferase (VTE2), dimethyl-phytylquinol methyl transferase (VTE3), tocopherol cyclase (VTE1) and γ-tocopherol C-methyl transferase (VTE4) are in blue types. Precursors and intermediates are: homogentisate (HGA), phytyl 2P (PDP), methyl-phytylquinol (MPBQ) and dimethyl-phytylquinol (DMPBQ). ( b ) Composition and total tocopherol contents (mean ±s.e.m, n =4) in ripe tomato fruits from the two parental species; S. lycopersicum (cv. M82) and S. pennellii (LA716), and the IL9-2-6 that shows the mapped QTL. ( c ) Fine mapping of the QTL 9-2-6 to a centromeric region of chromosome 9 harbouring the wild allele of VTE3 (1) gene. Through the analysis of 190 F2 and 50 F3 plants, derived from a cross between the S. lycopersicum (cv. M82) and the IL9-2-6, a recombinant subline (IL9-2-6-1) was obtained. Tocopherol contents (mean ±s.e.m, n =6) in ripe tomato fruits from these lines are shown on the right side of this panel. Genomic structure of the introgression contained in this line is shown below with black arrows indicating transcriptionally active genes. A magnified view of S. lycopersicum and S. pennellii alleles of VTE3 (1) gene shows synonymous (blue bars) and non-synonymous (red bar) polymorphisms and insertions in the second intron and in the 3′UTR. Black and grey boxes represent exons and, 5' and 3' UTR, respectively. ( d ) Protein structure of the tomato VTE3(1) enzyme indicating the amino acid substitution (S37P). ( e ) Transient expression of both alleles of VTE3(1)::GFP fusion protein in mesophyll cells of N. benthamiana leaves indicates chloroplast targeting under confocal microscopy examination. Asterisks in panels b and c denote statistically significant differences for total tocopherol (T) and the indicated tocopherol forms ( t -test P< 0.05). Scheme of chromosome 9 is based on physical distances calculated according to version SL2.4 of the tomato genome ( www.solgenomics.net ). White bar in e indicates 25 μm. Full size image The importance of tocopherol for both producer and consumer organisms has led to survey for quantitative trait loci (QTL) determining VTE content [3] , [12] , [13] , [14] , [15] . In tomato, we revealed the existence of four metabolic QTL (mQTL) affecting total tocopherol levels in fruits [9] . These four mQTL map onto chromosomes 6, 8 and 9. However, given the very low heritability (H 2 ) of VTE content in tomato [16] it will be difficult to breed fruit with elevated VTE contents until the genetic determinants and mechanisms underlying these QTL are fully understood. In this work, we report the fine mapping of the major VTE mQTL (mQTL 9-2-6 ) in tomato to a locus encoding a VTE3 enzyme. We show that VTE3(1) alleles are differentially expressed and that these differences correlate with differences in DNA methylation of the promoter sequences and in the accumulation of matching short interfering RNA (siRNAs). Consistent with mQTL 9-2-6 being of an epigenetic nature, we find that DNA methylation at VTE3(1) varies considerably among natural tomato populations and that VTE3(1) can spontaneously revert from methylated to unmethylated forms, with an impact on VTE contents in fruits. Fine mapping of a major tocopherol mQTL in tomato fruits We set out to identify the causal gene(s) harboured by the fruit-specific mQTL for total- and α-tocopherol contents that had previously been mapped to chromosome 9 (mQTL 9-2-6 ) [9] ( Fig. 1b and Supplementary Fig. 1a ). To this end, fine mapping was carried out using an F2 population of 190 individuals, derived from a cross between the parental S. lycopersicum line (cv. M82) and the introgressed line 9-2-6 (IL9-2-6) (spanning approximately 3 Mb and containing in excess of approximately 300 genes). The molecular markers C2_At3g63190 (58.9 Mb), VTE3(1)INDEL (59.6 Mb), C2_At4g02580 (60 Mb), 1531800 (61.0 Mb) and C2_At2g47890 (61.8 Mb) ( Supplementary Fig. 1b ) were used for screening and the introgressed fragment segregated 2:1:1 ( S.lyc / S.pen : S.lyc / S.lyc : S.pen / S.pen , χ 2 =0.98). A single recombinant line between C2_At4g02580 and 1531800 markers was identified and selfed to give rise to recombinant IL9-6-2-1, which harbours only 769 Kb of the original introgressed fragment. VTE quantification demonstrated that the total tocopherol mQTL was maintained in this recombinant IL ( Fig. 1c ). Out of the 56 putative Open reading frames (ORFs) present in this 789 Kb interval ( www.solgenomics.net ) 13 ORFs are not supported by any available expression data (expressed-sequence-tags or RNA-seq reads) and only 36 show detectable expression levels in tomato fruits. A MapMan [17] functional annotation analysis revealed that out of these 36, only a single gene ( VTE3 (1)-Solyc09g065730 locus-), belongs to the Secondary Metabolism category ( Supplementary Table 1 ). This gene displayed high similarity (~85%) to a dimethyl-phytylquinol methyl transferase from Arabidopsis (EC 2.1.1.-; Supplementary Fig. 1c,d ) that catalyses the conversion of 2-methyl-6-phytylquinol to 2,3-dimethyl-5-phytylquinol, the immediate precursor of γ-tocopherol ( Fig. 1a ) [18] . This gene is duplicated in several eudicot species including S. lycopersicum ( Supplementary Fig. 1c ). The tomato VTE3(1) has 339 amino acids and contains the two characteristic functional domains found in the Arabidopsis protein as well as a putative chloroplast transit peptide. When comparing the allelic divergence between the S. lycopersicum and S. pennellii proteins, a single amino acid polymorphism located within a lowly conserved region of the chloroplast transit peptide was found ( Fig. 1d and Supplementary Fig. 1d ). Transient subcellular localization assays performed with S. lycopersicum and S. pennellii alleles fused to GFP indicated that both VTE3(1) alleles are targeted to the chloroplast where tocopherol biosynthesis takes place ( Fig. 1e ). Taken together, these results suggest that VTE3 (1) is a major determinant of the mQTL 9-2-6-1 for fruit tocopherol content but that the causal polymorphism(s) are unlikely to reside within the coding sequence. VTE3 (1) mRNA levels modulate VTE contents in tomato fruits In order to demonstrate the involvement of VTE3 (1) in the determination of fruit tocopherol contents, we specifically silenced this gene in fruits by means of an established virus-induced gene silencing protocol, which relies on GFP fluorescence as a visual marker [19] . For this purpose a 380 bp fragment of the GFP coding region was fused to a 349 bp fragmentinsp of the VTE3 (1) tomato gene for cosilencing. Following the infiltration of inflorescent peduncles, fruit GFP -silenced sectors were monitored in planta across development and mature green (MG) and ripe tomatoes were harvested 42 and 60 days after infiltration, respectively. Sectors lacking fluorescence were dissected ( Fig. 2a ) and the levels of VTE3 (1) mRNA were measured by quantitative PCR (qPCR). Reductions of approximately 60% were observed in the GFP -silenced pericarp sectors with respect to fruits set from plants infiltrated with pTRV2-GFP alone ( Fig. 2b ). We next assayed the effect of VTE3 (1) silencing on fruit tocopherol metabolism. VTE3-dependent tocopherol forms (γ and α) showed significant reductions in both developmental stages, while VTE3-independent forms (δ and β) were increased more than twofold. Moreover, absolute levels of α- and γ-tocopherol were significantly reduced in VTE3 (1) silenced ripe fruits ( Fig. 2c ). These alterations in tocopherol metabolism were specifically related to VTE3 (1) silencing since mRNA levels of the other genes of the tocopherol core biosynthetic pathway ( VTE1 , VTE3 (2) and VTE4 ) were unaltered in this experiment ( Supplementary Fig. 2a ). Furthermore, a metabolic profiling analysis of the silenced tissues revealed no major alterations suggesting that this enzyme does not affect primary metabolism. However, increases in lycopene and α-carotene were detected in ripe fruits in which VTE3 (1) gene had been silenced ( Supplementary Fig. 2b ) and these changes were accompanied by an increased antioxidant capacity ( Supplementary Fig. 2c ). These data thus demonstrate that the alteration of VTE3 (1) mRNA levels directly affects tocopherol content and composition in tomato fruit and furthermore supports earlier hypotheses that fruit redox status is balanced by mechanisms which impact the metabolic pathways associated with both tocopherol and carotenoid metabolism [20] , [21] , [22] . 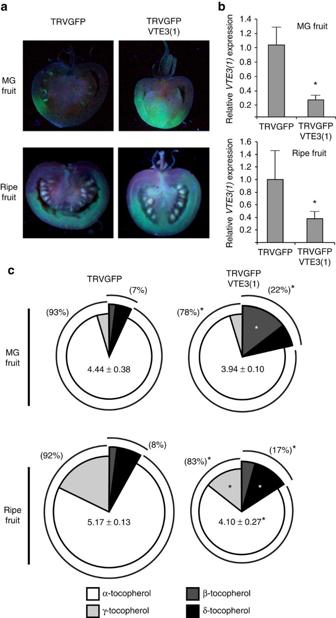Figure 2: Tocopherol contents inVTE3(1) transiently silenced tomato fruits. (a)GFP(control) andGFP-VTE3(1) silenced MG and ripe fruits harvested from virus-induced gene silencing agroinfiltrated inflorescent peduncles of GFP-expressing tomato plants (S. lycopersicumcv. Moneymaker). (b) Relative levels ofVTE3(1) mRNA inGFP(control) andGFP-VTE3(1) silenced fruits (mean ±s.e.m,n=6). (c) Tocopherol contents (μg g−1FW ±s.e.m,n=6), relative tocopherol composition and proportion of VTE3-dependent and VTE3-independent tocopherol forms from the same silenced fruits showed inaare indicated by numbers, pie charts and semicircles, respectively. Note that sizes of pie charts are proportional to the mean total tocopherol content. Asterisks denote statistically significant differences (t-testP<0.05). Figure 2: Tocopherol contents in VTE3 (1) transiently silenced tomato fruits. ( a ) GFP (control) and GFP - VTE3 (1) silenced MG and ripe fruits harvested from virus-induced gene silencing agroinfiltrated inflorescent peduncles of GFP-expressing tomato plants ( S. lycopersicum cv. Moneymaker). ( b ) Relative levels of VTE3 (1) mRNA in GFP (control) and GFP - VTE3 (1) silenced fruits (mean ±s.e.m, n =6). ( c ) Tocopherol contents (μg g −1 FW ±s.e.m, n =6), relative tocopherol composition and proportion of VTE3-dependent and VTE3-independent tocopherol forms from the same silenced fruits showed in a are indicated by numbers, pie charts and semicircles, respectively. Note that sizes of pie charts are proportional to the mean total tocopherol content. Asterisks denote statistically significant differences ( t -test P< 0.05). Full size image Specific VTE3 (1) alleles expression determines mQTL 9-2-6 Having demonstrated that VTE3 (1) expression determines tocopherol levels both at MG and ripe stages, we next compared the expression of the cultivated and wild alleles. In agreement with the tocopherol content profiles ( Fig. 1b ), the wild allele displayed significantly higher mRNA levels in ripe fruits from both introgression lines (IL9-2-6 and 9-2-6-1) in comparison with the recipient parental control. In other words, QTL 9-2-6 is an expression QTL (eQTL; Fig. 3a ). The higher mRNA accumulation of VTE3 (1) following introgression of the wild allele into the S. lycopersicum background was not restricted to mature fruits but was also observed in leaves and across fruit development ( Fig. 3b ). Moreover, these differences in VTE3 (1) expression are not accompanied by changes in the expression level of any of the other genes encoding the enzymes involved in the tocopherol biosynthetic pathway ( Fig. 3c ). Furthermore, evaluation of expression levels of 19 other ORFs present in the introgressed IL9-2-6-1 segment by qPCR showed similar results as those deposited in public data bases (ted.bti.cornell.edu), except for three ORFs. However, none of these three ORFs are known to be related to the VTE metabolism pathways and their expression does not correlate with tocopherol levels in tomato fruit. Also, the three A. thaliana orthologs are not coexpressed with any gene involved in the tocopherol biosynthesis [23] . Taken together, these results further confirm that VTE3(1) is the causal gene harboured by mQTL 9-2-6. 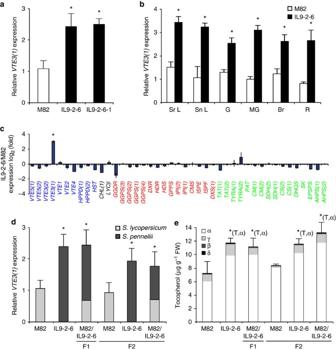Figure 3: An eQTL ofVTE3(1) is revealed in the tocopherol QTL9-2-6. (a)VTE3(1) mRNA levels in ripe fruits from the parental linesS. lycopersicum(cv. M82) and IL9-2-6 and the resulting recombinant IL9-2-6-1 (mean ±s.e.m,n=5). (b)VTE3(1)mRNA levels in source (Sr L) and sink leaves (Sn L) and along fruit development (green-G, mature green-MG, breaker-Br and ripe-R fruits) harvested from the parental linesS. lycopersicum(cv. M82) and IL9-2-6 (mean ±s.e.m,n=6). (c) mRNA levels quantified in ripe fruits from the parental linesS. lycopersicum(cv. M82) and IL9-2-6 of all genes encoding enzymes involved in tomato tocopherol metabolism according to24(mean ±s.e.m,n=3). Genes belonging to tocopherol core, associated, methylerythritol phosphate and shikimate pathways are indicated in blue, black, red and green, respectively. (d,e)VTE3(1) mRNA, tocopherol composition and total levels measured inVTE3(1) homozygous and heterozygous lines for two generations (F1 and F2) derived from a cross betweenS. lycopersicum(cv. M82) and IL9-2-6 (mean ±s.e.m,n=5). The contribution of eachVTE3(1) allele (S. lycopersicumandS. pennellii) was quantified by allele-specific quantitative reverse transcriptase-PCR and indicated by light and dark grey bars, respectively. Asterisks ina,b,candddenote statistically significant differences, (randomization testP<0.05 corrected by false discovery rate in case of multiple testing). Asterisks inedenote statistically significant differences for total tocopherol (T) and the indicated tocopherol forms (t-testP<0.05). Figure 3: An eQTL of VTE3 (1) is revealed in the tocopherol QTL 9-2-6 . ( a ) VTE3 (1) mRNA levels in ripe fruits from the parental lines S. lycopersicum (cv. M82) and IL9-2-6 and the resulting recombinant IL9-2-6-1 (mean ±s.e.m, n =5). ( b ) VTE3(1) mRNA levels in source (Sr L) and sink leaves (Sn L) and along fruit development (green-G, mature green-MG, breaker-Br and ripe-R fruits) harvested from the parental lines S. lycopersicum (cv. M82) and IL9-2-6 (mean ±s.e.m, n =6). ( c ) mRNA levels quantified in ripe fruits from the parental lines S. lycopersicum (cv. M82) and IL9-2-6 of all genes encoding enzymes involved in tomato tocopherol metabolism according to [24] (mean ±s.e.m, n =3). Genes belonging to tocopherol core, associated, methylerythritol phosphate and shikimate pathways are indicated in blue, black, red and green, respectively. ( d , e ) VTE3 (1) mRNA, tocopherol composition and total levels measured in VTE3 (1) homozygous and heterozygous lines for two generations (F1 and F2) derived from a cross between S. lycopersicum (cv. M82) and IL9-2-6 (mean ±s.e.m, n =5). The contribution of each VTE3 (1) allele ( S. lycopersicum and S. pennellii ) was quantified by allele-specific quantitative reverse transcriptase-PCR and indicated by light and dark grey bars, respectively. Asterisks in a , b , c and d denote statistically significant differences, (randomization test P< 0.05 corrected by false discovery rate in case of multiple testing). Asterisks in e denote statistically significant differences for total tocopherol (T) and the indicated tocopherol forms ( t -test P< 0.05). Full size image To further unravel the nature of the VTE3 (1) eQTL, its transgenerational stability was analysed in ripe fruits from the F1 hybrid and F2 segregating lines with the three possible allele combinations determined by an allele-specific expression assay. In the F1 hybrid, the total VTE3 (1) mRNA level is equivalent to that measured in IL9-2-6 as a consequence of the dominance of the wild allele. Similarly, VTE3 (1) expression displays the same pattern in the derived F2 recombinant lines ( Fig. 3d ). Moreover, the total tocopherol content follows the same profile as that of the VTE3 (1) mRNA levels ( Fig. 3e ), suggesting that the mQTL 9-2-6 and the VTE3 (1) eQTL are tightly and stably coupled across generations. Revealing the molecular mechanism of the tocopherol QTL 9-2-6 The higher VTE3 (1) mRNA levels in IL9-2-6 and IL9-2-6-1 could be the result of differences in the transcriptional promoter activities between the domesticated and wild alleles. Therefore, we analysed the promoter regions of these alleles by a de novo search for cis -regulatory elements (CREs) [24] . The S. lycopersicum VTE3 (1) gene promoter contains seven statistically overrepresented CREs, while the S. pennellli one contains four. Two of these elements are common to the S. lycopersicum , S. pennellii and S. phureja VTE3 (1) promoter regions ( Supplementary Fig. 3a ). Further comparisons between the promoter regions of S. lycopersicum , S. pimpinellifolium , S. pennellii and S. phureja revealed distinct patterns of transposable element (TE) insertions. While two copies of the Tc1-IS630-Pogo family of DNA transposons [25] are common between all four analysed species, indicating that they were present in the common ancestral, a retrotransposon element of the SINE family [26] is exclusively found in the closest species S. lycopersicum and S. pimpinellifolium , suggesting a later specific insertion in the tomato lineage (section Lycopersicon; Supplementary Fig. 3b ). Furthermore, the genomic region spanning this SINE is highly methylated in fruits from S. lycopersicum (cv Ailsa Craig) ( http://ted.bti.cornell.edu/epigenome/ ), mainly at CHH sites, which is a hallmark of RNA-directed DNA methylation (RdDM) [27] . In order to address whether the RdDM machinery may be involved in the establishment and maintenance of the DNA methylation in this region, we next generated siRNA-seq profiles from ripe fruits of S. lycopersicum, S. pennellii and the IL9-2-6-1. We found that a considerable number of 21-24 nt-siRNAs species (sense and antisense) matches the TE sequences located in the promoter of S. lycopersicum ( Fig. 4a,b ), but none in S. pennellii nor in the IL9-2-6-1. By means of McrBC enzyme digestion and allele-specific semiquantitative PCR, we assessed the methylation status of three different fragments of VTE3 (1) gene: two on the promoter region (I and II) and one on the coding sequence (III). The results revealed that the proximal promoter region of S. lycopersicum allele harbouring the SINE TE is hypermethylated, whilst the wild one, either in its own background ( S. pennellii ) or in the M82 background (IL9-2-6 and IL9-2-6-1), showed low levels of DNA methylation ( Fig. 4c ). To better characterize these epialleles, we investigated DNA methylation at single-nucleotide resolution, using bisulphite treatment of genomic DNA followed by targeted sequencing. Results confirmed hypermethylation of the proximal VTE3 (1) promoter region (II) of the S. lycopersicum allele in the three genomic contexts ( Fig. 4d ). Since siRNAs seem to be involved in the establishment of the hypermethylated epiallele of VTE3 (1), we tested the existence of allelic interactions such as paramutation [28] . To determine whether this is the case or not, we next analysed the allele-specific DNA methylation in the F1 hybrids and F2 heterozygous. In line with the expression results ( Fig. 3d ), we found that the epigenetic status of each allele remains unaltered in the hybrids, demonstrating that they are not targets of paramutation ( Supplementary Fig. 4 ). 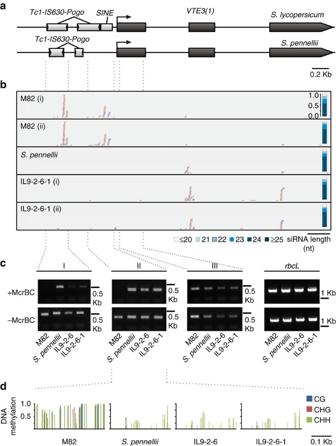Figure 4: siRNA profile and methylation status of the wild and cultivated alleles ofVTE3(1) gene. (a)VTE3(1) gene and promoter structure (4 Kb window) showing exons (black boxes) and TE insertions (light grey boxes). (b) Locus-specific siRNA profiles of theVTE3(1). Tracks show mapping position of sense (red) and antisense (blue) unique siRNA obtained from ripe fruits ofS. lycopersicum(cv. M82),S. pennellii(LA716) and IL9-2-6-1. The length distribution of the mapped siRNAs is represented on the right of each track. siRNA fromS. lycopersicum(cv. M82) and IL9-2-6-1 were extracted and analysed from two pools of fruits harvested from independent plants (indicated by i and ii), while fromS. pennellii(LA716) were extracted and analysed from a pool of five fruits. (c) DNA methylation status assayed by a McrBC methylation-sensitive endonuclease DNA treatment followed by PCR amplification in two regions of theVTE3(1) promoter (I: distal and II: proximal), in the first exon of the gene (III) and on a coding region of the Rubisco LS chloroplast gene (rbcL) as a control. DNA was extracted from at least four ripe fruits of theS. lycopersicum(cv. M82),S. pennellii(LA716), IL9-2-6 and IL9-2-6-1 genotypes. (d) Methylation of cytosine residues in CG, CHG and CHH sites (blue, red and green lines, respectively) assayed by bisulphite sequencing of the proximal promoter region (region II in c) in DNA extracted from ripe fruits of theS. lycopersicum(cv. M82),S. pennellii(LA716), IL9-2-6 and IL9-2-6-1 genotypes. Figure 4: siRNA profile and methylation status of the wild and cultivated alleles of VTE3 (1) gene. ( a ) VTE3 (1) gene and promoter structure (4 Kb window) showing exons (black boxes) and TE insertions (light grey boxes). ( b ) Locus-specific siRNA profiles of the VTE3(1) . Tracks show mapping position of sense (red) and antisense (blue) unique siRNA obtained from ripe fruits of S. lycopersicum (cv. M82), S. pennellii (LA716) and IL9-2-6-1. The length distribution of the mapped siRNAs is represented on the right of each track. siRNA from S. lycopersicum (cv. M82) and IL9-2-6-1 were extracted and analysed from two pools of fruits harvested from independent plants (indicated by i and ii), while from S. pennellii (LA716) were extracted and analysed from a pool of five fruits. ( c ) DNA methylation status assayed by a McrBC methylation-sensitive endonuclease DNA treatment followed by PCR amplification in two regions of the VTE3 (1) promoter (I: distal and II: proximal), in the first exon of the gene (III) and on a coding region of the Rubisco LS chloroplast gene ( rbcL ) as a control. DNA was extracted from at least four ripe fruits of the S. lycopersicum (cv. M82), S. pennellii (LA716), IL9-2-6 and IL9-2-6-1 genotypes. ( d ) Methylation of cytosine residues in CG, CHG and CHH sites (blue, red and green lines, respectively) assayed by bisulphite sequencing of the proximal promoter region (region II in c) in DNA extracted from ripe fruits of the S. lycopersicum (cv. M82), S. pennellii (LA716), IL9-2-6 and IL9-2-6-1 genotypes. Full size image In order to evaluate whether the methylation-dependent regulation of the S. lycopersicum VTE3 (1) allele is an M82-specific mechanism or rather one that can be extended to other genetic backgrounds, we further analysed the expression of VTE3 (1) and DNA methylation across an allelic series of tomato Andean landraces, three commercial reference cultivars and one closely ( S. pimpinellifolium -LA1589) and one distantly related wild species ( S. habrochaites -LA407). These accessions were collected from different geographical locations and assayed under the same field conditions. Previously published results demonstrated that they differ in tocopherol and carotenoid contents [24] . We found that both VTE3 (1) expression and methylation of its proximal promoter region vary among the different genotypes. Furthermore, VTE3 (1) mRNA abundance inversely correlates with the methylation levels of the proximal promoter region ( Fig. 5a and Supplementary Fig. 5a ). Accordingly, the cultivars with higher VTE3 (1) mRNA levels accumulate more γ-tocopherol in mature fruits ( Supplementary Fig. 5b ). Sequence analysis of a 850 bp interval encompassing the promoter of VTE3 (1) gene from the 13 genotypes studied here revealed the presence of single-nucleotide polymorphisms and small InDels, but these do not correlate with differences in expression level or DNA methylation ( Supplementary Figs 5a and 6 ). 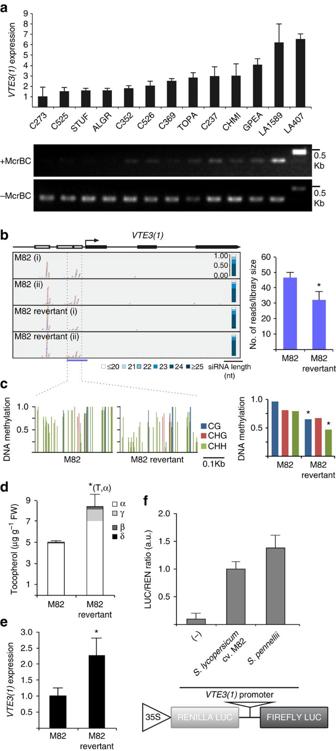Figure 5: Natural occurring epiallele regulatesVTE3(1) gene expression and tocopherol levels. (a)VTE3(1) mRNA levels (mean ±s.e.m,n=3) and DNA methylation status assayed by a McrBC methylation-sensitive endonuclease DNA treatment, followed by PCR amplification of the proximal promotor region (analysed inFig. 4d) in ripe fruits from eight tomato Andean landrace (S. lycopersicum), three commercial reference cultivars and the wild speciesS. pimpinellifolium(LA1589) andS. habrochaites(LA407). (b) Locus-specific siRNAs profiles ofVTE3(1). Tracks show mapping position of sense (red) and antisense (blue) unique siRNA from ripe fruits harvested fromS. lycopersicum(cv. M82) cultivated under greenhouse conditions and from a field trial performed in Mendoza (Argentina, 32° 50′S, 68° 52′W and 900 masl). The length distribution of the mapped siRNAs is represented on a box at the right of each track. The bar plot on the right panel shows the normalized number (±s.e.m,n=2) of siRNAs mapped on the proximal promoter region ofVTE3(1)(indicated by a blue line below the tracks panel). siRNAs were extracted and analysed from two pools of fruits harvested from independent plants each (indicated by i and ii) (c) Methylation of cytosine residues in CG, CHG and CHH sites (blue, red and green lines, respectively) assayed by targeted bisulphite sequencing of the proximal promoter region (analysed inFig. 4d) from DNA extracted from a pool of the same samples as inb. The bar plot on the right panel shows the quantification of DNA methylation for each context. (d,e) Tocopherol composition andVTE3(1) mRNA levels (mean ±s.e.m,n=3) from the same samples as inbandc. (e) Transcriptional activity of wild and cultivated allele promoters measured by a transient assay using the pGreenII 0800-LUC vector as described in the Methods (±s.e.m,n≥6). Asterisk in panelb,candedenotes statistically significant differences (t-test, Fisher test and randomization test, respectively;P<0.05). Asterisk inddenotes statistically significant differences for total tocopherol (T) and the indicated tocopherol forms (t-testP<0.05). Figure 5: Natural occurring epiallele regulates VTE3 (1) gene expression and tocopherol levels. ( a ) VTE3 (1) mRNA levels (mean ±s.e.m, n =3) and DNA methylation status assayed by a McrBC methylation-sensitive endonuclease DNA treatment, followed by PCR amplification of the proximal promotor region (analysed in Fig. 4d ) in ripe fruits from eight tomato Andean landrace ( S. lycopersicum ), three commercial reference cultivars and the wild species S. pimpinellifolium (LA1589) and S. habrochaites (LA407). ( b ) Locus-specific siRNAs profiles of VTE3(1) . Tracks show mapping position of sense (red) and antisense (blue) unique siRNA from ripe fruits harvested from S. lycopersicum (cv. M82) cultivated under greenhouse conditions and from a field trial performed in Mendoza (Argentina, 32° 50′S, 68° 52′W and 900 masl). The length distribution of the mapped siRNAs is represented on a box at the right of each track. The bar plot on the right panel shows the normalized number (±s.e.m, n =2) of siRNAs mapped on the proximal promoter region of VTE3(1) (indicated by a blue line below the tracks panel). siRNAs were extracted and analysed from two pools of fruits harvested from independent plants each (indicated by i and ii) ( c ) Methylation of cytosine residues in CG, CHG and CHH sites (blue, red and green lines, respectively) assayed by targeted bisulphite sequencing of the proximal promoter region (analysed in Fig. 4d ) from DNA extracted from a pool of the same samples as in b . The bar plot on the right panel shows the quantification of DNA methylation for each context. ( d , e ) Tocopherol composition and VTE3 (1) mRNA levels (mean ±s.e.m, n =3) from the same samples as in b and c . ( e ) Transcriptional activity of wild and cultivated allele promoters measured by a transient assay using the pGreenII 0800-LUC vector as described in the Methods (±s.e.m, n ≥6). Asterisk in panel b , c and e denotes statistically significant differences ( t -test, Fisher test and randomization test, respectively; P< 0.05). Asterisk in d denotes statistically significant differences for total tocopherol (T) and the indicated tocopherol forms ( t -test P< 0.05). Full size image Finally, we found that the number of siRNAs targeting the SINE element and the methylation status of the VTE3 (1) promoter reverted when the reference cultivar M82 (the recurrent parental line of the ILs) was grown under field conditions ( Fig. 5b,c ). This epiallelic conversion was accompanied by an increase in the level of VTE3 (1) mRNA as well as in the levels of tocopherol in ripe fruits ( Fig. 5d,e ). These results provide therefore conclusive evidence of the epigenetic nature of mQTL 9-2-6 . Moreover, when the transcriptional activity of the two de-methylated promoters was tested in a transient expression assay no differences were detected ( Fig. 5f ), demonstrating that the difference in VTE3 (1) expression of both alleles results from the specific epigenetic silencing of the S. lycopersicum variant. When taken in combination, the sum results presented here demonstrate that S. pennellii and S. lycopersicum VTE3 (1) are epialleles and strongly hint that their differential behaviour is determined by the presence of TE insertions within the promoter region. Identification of genes that impact on the nutritional quality of domesticated fruits and vegetables has been a major goal of modern breeding programs. Cultivated tomato is one of the most consumed vegetables in the world and because of the relatively high levels of tocopherol found in tomato fruits, this vegetable is an important source of VTE in the human diet [7] . However, it has been documented that VTE content is a low heritability trait [16] , therefore a more comprehensive knowledge of the genetic factors underlying this trait is a prerequisite for nutritional quality improvement. In this work, we focused on a major mQTL for total tocopherol, which maps to the introgressed region of the S. pennellii IL9-2-6 and explains about 50% of the variation in VTE between the parental genotypes. By means of a fine mapping approach we were able to restrict the genetic determinant of the mQTL 9-2-6 to a pericentromeric region of chromosome 9 harbouring the VTE3 (1) locus. This gene encodes a 2-methyl-6-phytylquinol methyl transferase which is a central enzyme for α-tocopherol and γ-tocopherol synthesis ( Fig. 1a ). VTE3 was the subject of an ancient duplication event that, according to the substitution rate calculated for tomato [29] , we estimated took place 152±24 Myr ago, following the radiation between eudicots and monocots. Comparison of the VTE3 (1) coding regions from S. pennellii and S . lycopersicum revealed a single non-synonymous substitution in a non-conserved region within the chloroplast transit peptide ( Fig. 1d and Supplementary Fig. 1d ), which does not impact protein targeting as indicated by GFP fusion experiments ( Fig. 1e ). Moreover, the virus-mediated transient silencing assay demonstrated that the alteration of VTE3 (1) mRNA levels directly affects tocopherol contents and composition in tomato fruit ( Fig. 2 ) and that this effect is likely due to a redirection of carbon flow from the α- and γ-tocopherol branch to the β- and δ-tocopherol branch of the pathway ( Fig. 1a ). Reductions in VTE3(1) activity would also likely result in an increase in the availability of geranylgeranyl 2P, a precursor of carotenoid biosynthesis. Accordingly, fruit tissues silenced for VTE3 (1) showed significant increments in lycopene and α-carotene levels and in the antioxidant capacity. The wild allele of VTE3 (1) displayed significantly higher mRNA levels in all tested organs and developmental stages, indicating the existence of an eQTL ( Fig. 3a,b ). Additional examination of hybrids (F1 and F2) derived from a cross between S. lycopersicum (cv. M82) and IL9-2-6, demonstrated that the wild allele is dominant and stable through generations. Moreover, the mQTL 9-2-6 co-varies with VTE3 (1) expression, suggesting that this eQTL determines VTE levels ( Fig. 3d,e ). Furthermore, VTE3 (1) upregulation in IL9-2-6 and IL9-2-6-1 favour carbon flow to α-tocopherol ( Fig. 1c ), supporting VTE3 (1) as the causal gene of the mQTL 9-2-6 . However, the absolute levels of the other tocopherol forms did not show significant differences. Because a second VTE3 gene copy is present in tomato (like in other higher plant species Supplementary Fig. 1c ) and many factors (for example, oxidative stress status) can significantly affect tocopherol content, either epistatic or pleiotropic effects cannot be discarded and should be considered for further studies. Several reports have linked eQTLs to phenotypic variation in plants [30] ; however, in tomato only a few has been proposed [31] , [32] , [33] . Further experimentation allowed us to uncover that VTE3 (1) eQTL is determined by differential methylation level of the wild and cultivated alleles. In addition, this differential epigenetic regulation is associated with a specific fragment within the regulatory region of VTE3 (1) that harbours a SINE TE that is present in only some species of the Lycopersicon section ( Supplementary Figs 3b and 6 ). Moreover, this TE insertion is predominantly methylated at CHH sites and matches with a considerable number of siRNAs ( Figs 4 and 5 ), suggesting the involvement of the RdDM machinery in the establishment and maintenance of DNA methylation at this locus [27] . Accordingly, the promoter of VTE3(1) lacks the SINE insertion and is unmethylated in S. pennellii. On the other hand, this SINE insertion is not always methylated when present in the promoter of VTE3(1) and conversion from the methylated to the unmethylated state was observed in some cases ( Fig. 5 and Supplementary Fig. 5 ). These results demonstrate that the mQTL 9-2-6 is of an epigenetic nature and that variation in caused by the differential methylation of the TE sequence located in the promoter region of the VTE3 (1) gene. To our knowledge, this is the first report unravelling an epigenetic QTL for a highly valuable nutritional trait. A small number of genes with natural epialleles leading to different phenotypes have been described in plants, which determine floral symmetry in Linaria vulgaris [34] , sex determination in melon [35] or plant stature in rice [36] . In tomato, epigenetic regulation has already been reported for the cnr (colourless non-ripening) locus encoding a SBP-box transcription factor, which results in ripening defective fruits. Interestingly, revertant ‘ripening’ sectors have been reported [37] , [38] . In this sense, epialelle reversion has been seen to be a common phenomenon in plants [39] , [40] , [41] . In addition, several epigenetic QTL for flowering time and root length have been mapped using an experimental population of isogenic A. thaliana that segregates induced DNA methylation changes [42] . Our results extend these findings by providing direct evidence for the existence of epigenetic QTL (QTL epi ) in natural populations. The existence of a second VTE3 copy in tomato might have been important for the establishment of the epiallelic variation at VTE3 (1), since the spontaneous downregulation of VTE3 (1) by methylation in S. lycopersicum could be compensated by the second copy, avoiding the deleterious phenotype of tocopherol reduction on seed longevity and stress response [11] . This situation is analogous to that underlying a case of genetic incompatibility in Arabidopsis [43] . Epigenetic-dependent gene expression regulation associated with the presence of TEs insertions has also been described. This is the case of FWA gene in Arabidopsis for which the transcription level depends on the methylation status of a SINE element contained in the promoter region [44] . Moreover, a genome wide study revealed that methylated TE insertions are frequently associated with reduced expression of adjacent genes, therefore being subject of purifying selection [45] . In this line, the presence of a SINE TE insertion on the promoter region of VTE3 (1) gene, which enables the existence of several epialleles in natural populations of tomatoes, determines tocopherol accumulation in fruit ( Fig. 5a ). Furthermore, the epigenetic regulation of tocopherol levels documented here might be suggesting a role of naturally occurring epialleles in heritable environmental adaptation. Probably because of their sessile nature, plants have extensively enhanced genetic and epigenetic strategies for coping with different environmental conditions. The tocopherol mQTL determined by epialleles allow us to extend this phenomenon to the tuning of antioxidant potential that might provide adaptation advantages. In light of the results presented here, the low heritability of the tocopherol content trait [16] can now be reinterpreted due to the epigenetic and reversible nature of mQTL 9-2-6 , where the instability of epialleles produce phenotypic dynamics that cannot be predicted from strictly Mendelian models of inheritance. Further studies aiming to understand the genetic determinants of other natural and low heritability traits will allow the development of a population genetics theory which will incorporate the epigenetic information and therefore be capable to predict plants phenotypes and their stabilities in a more accurate manner. Plant materials and growth conditions Tomato seeds from S. lycopersicum cv. M82 (LA3475), S. pennelli (LA716), IL9-2-6 (LA4083), were obtained from the Tomato Genetic Resource Center ( http://tgrc.ucdavis.edu ). S. lycopersicum cv. MoneyMaker-GFP#6 were obtained from ref. 19 . Nicotiana benthamiana seeds were obtained from Dr Roger Beachy (Stanford University, CA, USA). Tomato and N. benthamiana plants were grown in 20 l pots under greenhouse conditions: 16/8 h photoperiod, 24±3 °C, 60% humidity, and 300±100 μmol m −2 s −1 incident photoirradiance. Source (Sr L) and sink (Sn L) leaves were collected from 8-week-old plants. Fruits at green (G), MG, breaker (B) and ripe (R) stage were harvested 30, 45, 50 and 60 days after anthesis, respectively. Seeds of the eight Andean landrace cultivars, commercial reference cultivars (GPEA, ALGR and STUF) and the two wild species; S. pimpinellifolium (LA1589) and S. habrochaites (LA407), were obtained from the germoplasm bank of the EEA-INTA-La Consulta (Argentina). The last two accessions were reproduced from seeds originally sent by the Tomato Genetic Resource Center. Seedlings were grown until four true leaves in 150 ml pots and transplanted to soil under field-production conditions in the Campo Experimental del Instituto de Horticultura, Universidad Nacional de Cuyo, Mendoza, Argentina, 32° 50′S, 68° 52′W and 900 masl. The field experiment was conducted from October 2008 to March 2009 in a randomized design of three replicates with three plants each. The experiment was protected with an antihail mesh and crop irrigation was applied to keep soil available water content constant. At ripe stage, two fruits per plant were harvested approximately 60–65 days after anthesis and immediately frozen in liquid N 2 and kept at −80 °C until use. Tocopherol quantification by high-performance liquid chromatography Tocopherol extraction and quantification was performed exactly as previously described [9] . Briefly, tomato fruits were ground to a fine powder in liquid nitrogen and 500 mg of material was extracted with 1.5 ml methanol and, after vortex mixing, 1 ml chloroform was added. Following 5 min of sonication, 1 ml of Tris buffer (Tris (pH 7.5, 50 mM), NaCl 1 M) was added. The chloroform phase was recovered and the methanol phase (remaining pellet) was reextracted with chloroform (2 ml). Chloroform extracts were pooled and adjusted to a final volume of 4 ml. Two ml were dried under nitrogen gas and resuspended in 0.2 ml of 99.5:0.5 hexane:isopropanol. The tocopherol content was determined using a Hewlett-Packard series 1100 HPLC system coupled with a fluorescence detector (Agilent Technologies series 1200). Separation was carried out on a normal-phase column Metasil Si (250 mm × 4.6 mm, 5 μm, Varian, Metachem, Torrance, CA) maintained at room temperature using a isocratic solvent system (mobile phase) consisting of 99.5:0.5 hexane/isopropanol with a flow rate at 1 ml min −1 . Eluting compounds were detected and quantified by fluorescence with excitation at 296 nm and emission at 340 nm. Identification and quantification of tocopherol compounds was achieved by comparison with the retention times and peaks areas of standards purchased from Merck (tocopherol set Calbiochem #613424). A daily calibration curve was carried out using a tocopherol solution with a concentration range between 0.31 and 5 μg ml −1 for each isoform. Fine mapping of the tocopherol QTL 9-2-6 Flowering plants from the S. lycopersicum cv. M82 and from the IL9-2-6 were crossed. F1 hybrid was selfed and 190 F2 and 50 F3 plants were screened with five codominants molecular markers distributed along the introgression: PCR-markers C2_At3g63190 and C2_At2g47890, and the CAP-marker C2_At4g02580 were obtained from http://solgenomics.net . VTE3(1)INDEL (Chr.9: 59.6 Mb) and 1531800 (Chr.9: 61.0 Mb) markers were designed based on InDels identified between S. lycopersicum and S. pennellii VTE3 (1) allele's sequences and a flanking region, respectively. An F2 plant recombinant between C2_At4g02580 and 1531800 markers was selfed and the homozygous lines IL9-2-6-1 was selected from the F3 population. Primer sequences are listed in Supplementary Table 2 . VTE3 (1) subcellular localization The full lenght cDNA of both alleles of VTE3 (1) was amplified by PCR using Taq Platinum Pfx DNA polymerase (Invitrogen) and cloned into the binary vector pK7FWG2 by recombination using LR clonase (Invitrogen) resulting in a C-terminal green fluorescent protein (GFP) fusion protein (pK7FWG2-VTE3(1)). Primer sequences are listed in Supplementary Table 2 . Transient expression via Agrobacterium tumefaciens and confocal microscopy examination were performed as has been previously described [46] . Virus-induced gene silencing of VTE3 (1) Construct, infiltration and fruit harvesting procedures were performed as has been previously described [19] . Briefly, a 349-bp fragment of the VTE3(1) gene (Solyc09g065730) was amplified from tomato leaves cDNA (primer sequences are listed in Supplementary Table 2 ) and cloned into the pTOPO 2.1 vector (Invitrogen) giving rise to the pTOPO-VTE3.1 vector. pTOPO- gfp 380 (ref. 19 ) and pTOPO-VTE3.1 vectors were digested with EcoRI restriction enzyme (NEB) and ligated at room temparature for 2 h using 0.4 unit of T4 DNA Ligase (NEB). Ligation products were subsequently amplified by PCR and a 729 bp PCR product were inserted into the pCR8/GW/TOPO vector (Invitrogen). The resulting vectors were recombined into the pTRV2-GW vector [19] . pTRV1, pTRV2-GFP [19] and pTRV2-GFP-VTE3(1) were introduced into Agrobacterium tumefaciens strain GV3101. A 5-ml culture was grown overnight at 28 °C in 50 mg l −1 gentamycin and 50 mg l −1 kanamycin in LB medium and used to inoculate 50 ml of LB medium containing the same antibiotics. After an overnight culture at 28 °C, cells were harvested by centrifugation and resuspended in infiltration media (10 mM MgCl 2 , 10 mM MES and 200 mM acetosyringone), adjusted to an OD600 of 1.0, and left at room temperature for 4 h. Equivalent aliquots of GV3101-pTRV1 and -pTRV2 were mixed immediately before inoculation. One week preanthesis inflorescence peduncles of 8-week-old tomato plants were wounded with a needle (27 G ½ inches) and approximately 40 μl of the Agrobacterium suspension was delivered. Pericarp tissue from MG and ripe fruits were harvested 42 and 60 days after infiltration, respectively. All samples were immediately frozen in liquid N 2 and stored at −80 °C until use. RNA isolation and qPCR analysis Total RNA was extracted from 50 mg and 100 mg of frozen leaves and fruit pericarps, respectively, with TRIZOL reagent (Invitrogen) according to the manufacturer’s instructions. DNA traces were removed by treatment with amplification-grade DNAse I (Invitrogen) following the manufacturer’s instructions. cDNA was synthesized from 1 μg of total RNA using random primers and the SuperScript III enzyme (Invitrogen) in a final volume of 20 μl. Reactions were carried out in duplicate using 2X SYBR Green Master Mix reagent (Applied Biosystems) in a 20 μl final volume and a 7500 real-time PCR system (Applied Biosystems). Primers used for gene expression analysis of VTE3 (1) and the 19 selected ORFs spanning on the IL9-2-6-1 introgressed fragment are listed in Supplementary Table 2 . Primer sequences for VTE biosynthetic pathway enzymes encoding genes were as previously described [24] and are included in Supplementary Table 2 . Gas chromatography-mass spectrometry Metabolites extraction and quantification was performed exactly as described before [19] . Briefly, tomato frozen tissues (~ 250 mg) were extracted with 2000 μl of methanol and 120 μl of internal standard (0.2 mg ml −1 water of ribitol) was added for quantification. The mixture was extracted for 15 min at 70 °C, mixed vigorously with one volume of water, centrifuged at 2,200 g and subsequently reduced to dryness under vacuum. The residue was redissolved and derivatized for 120 min at 37 °C (in 60 μl of 30 mg ml −1 methoxyamine hydrochloride in pyridine) followed by a 30-min treatment at 37 °C with 120 μl of N -methyl- N -[trimethylsilyl] trifluoroacetamide. Sample volumes of 1 μl were then injected in splitless and split modes, using a hot needle technique. The gas chromatography–time-of-flight–mass spectrometry (GC-tof-MS) system was composed of an AS 2000 autosampler, a GC 6890N gas chromatographer (Agilent Technologies, USA), and a Pegasus III time-of-flight mass spectrometer (LECO Instruments, USA). Mass spectra were recorded at 20 scans s −1 with a scanning range of 70 to 600 m/z. Both chromatograms and mass spectra were evaluated using ChromaTOF chromatography processing and mass spectral deconvolution software, version 3.00 (LECO Instruments, USA). Identification and quantification of the compounds were performed with TagFinder 4.0 software [47] and the mass spectra were cross referenced with those in the Golm Metabolome Database [48] , [49] . Six biological replicates were used for this analysis. Promoter sequence analyses In silico CRE identification was performed as indicated [24] . TEs were identified by WU-BLAST (v4.0.3 version) with RepeatMasker [50] against the Solanacea database. McrBC-based methylation assay Genomic DNA was extracted from 100 mg of tomato fruits by PhytoPure kit (GE Healthcare). A quantity of 1 μg of DNA was digested for 3 h with 10 U of McrBC enzyme (NEB) in parallel with a mock reaction. 50 ng of digested DNA was further used for 28 cycles PCR amplifications in 1X reaction buffer with 0.75 mM MgCl2, 0.1 μM dNTPs, 0.4 μM primer concentration and 1 unit of Platinum TAQ DNA polymerase (Invitrogen). Cycling conditions were: 15 s 94 °C, 1 min 55 °C and 1 min 72 °C. Primer sequences are listed in Supplementary Table 2 . Bisulphite analysis Bisulphite treatment was performed on 200 ng of genomic DNA using the EZ DNA Methylation-Gold Kit (Zymo Reseacrh). The treated DNA was amplified by nested PCR using the primers listed in the Supplementary Table 2 . Amplified fragments were cloned into pGEM-T vector (Promega) for sequencing. At least nine clones of each genotype were sequenced. The bisulphite conversion efficiency was calculated by analysing a chloroplast loci [51] indicating a conversion rate greater than 99%. siRNA analysis Small RNAs from ripe fruits were extracted using mirVana Kit (Ambion) according to the manufacturer's instructions. RNA libraries were multiplexed and sequenced on a HiSeq2500 system (Illumina) obtaining ~12 million of high quality reads per library. After clipping with fastx_clipper (FASTX-Toolkit), reads were mapped without mismatches to the reference sequences of S. lycopersicum and S. pennellii VTE3 (1) loci using bowtie2 software [52] . Mapping visualization were carried on using Integrative Genomics Viewer (IGV) [53] . Small RNA sequence information is provided in Supplementary Table 3 . VTE3(1) promoter activity assay A promoter region of approximately 1000, bp from the two VTE3(1) alleles was cloned into the MCS upstream of the firefly luciferase (LUC) in the vector pGreenII 0800-LUC harbouring the Renilla luciferase (REN) gene under the control of the 35S promoter [54] , transformed into Agrobacterium tumefaciens cells (GV3101 strain) and infiltrated in fully expanded leaves of Nicotiana benthamiana adult plants. After 2 days, leaves were harvested and measured for LUC and REN activities by using the Dual-Luciferase Reporter Assay System (Promega). Accession codes. The siRNA sequencing data have been deposited in the ENA short read archive under project number PRJEB6247 and accessions codes ERR493820 to 93826. How to cite this article: Quadrana, L. et al. Natural occurring epialleles determine vitamin E accumulation in tomato fruits. Nat. Commun. 5:4027 doi: 10.1038/ncomms5027 (2014).